Multiple independent autonomous hydraulic oscillators driven by a common gravity head Self-switching microfluidic circuits that are able to perform biochemical experiments in a parallel and autonomous manner, similar to instruction-embedded electronics, are rarely implemented. Here, we present design principles and demonstrations for gravity-driven, integrated, microfluidic pulsatile flow circuits. With a common gravity head as the only driving force, these fluidic oscillator arrays realize a wide range of periods (0.4 s–2 h) and flow rates (0.10–63 μl min −1 ) with completely independent timing between the multiple oscillator sub-circuits connected in parallel. As a model application, we perform systematic, parallel analysis of endothelial cell elongation response to different fluidic shearing patterns generated by the autonomous microfluidic pulsed flow generation system. Although the electronic–fluidic analogy [1] , [2] is commonly inferred, microfluidic circuits that can simultaneously perform multiple independent parallel operations in an autonomous fashion have yet to be implemented. Constant-voltage electronic circuit designs allow instructions to be embedded in the arrangement of circuit components in a way that multiple tasks can be performed autonomously and independently in parallel ( Fig. 1a ). This enables electronic circuits to be automated and user-friendly while also being versatile and multifunctional. Microfluidic circuits, however, still require instruction from external controllers and do not demonstrate independent parallel processing capabilities. Even microfluidic logic circuits [3] , [4] , [5] , [6] , [7] generally require instruction from computer-programmed, time-varying input pressures and thus do not operate autonomously. Our previously described constant flow-driven oscillator circuits can generate pulsatile flows autonomously but cannot generate independent, parallel flows [8] , [9] , [10] , [11] . A fluidic astable multivibrator driven by a constant pressure source was described 20 years ago, but without multiplexing or application demonstrations [12] . 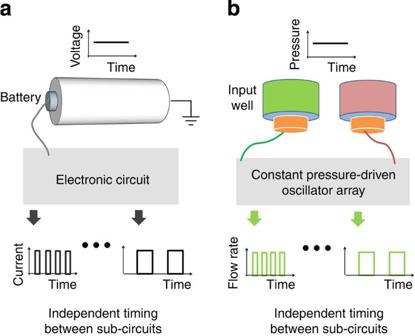Figure 1: Electronic–fluidic analogy of instruction-embedded oscillator arrays. (a) Electronic circuits with embedded instructions to perform multiple parallel operations with independent timing are typically driven by a constant-voltage source. (b) Hydraulic oscillator system described in this paper. This circuit has embedded instructions to produce multiple parallel periodic flows with different flow rates and independent timing using a constant gravitational potential as the driving fluid input source. Figure 1: Electronic–fluidic analogy of instruction-embedded oscillator arrays. ( a ) Electronic circuits with embedded instructions to perform multiple parallel operations with independent timing are typically driven by a constant-voltage source. ( b ) Hydraulic oscillator system described in this paper. This circuit has embedded instructions to produce multiple parallel periodic flows with different flow rates and independent timing using a constant gravitational potential as the driving fluid input source. Full size image Here, we describe microhydraulic circuits that implement autonomous and independent parallel flow-switching in a manner similar to capabilities of constant-voltage electronic circuits. Using a gravity water head (0.3–0.7 m) as the driving force, the circuits perform embedded instructions in multiple parallel sub-circuits ( Fig. 1b ). Our practical goal is to replace off-chip controllers [13] , [14] that generate time-varying input pressure with gravity-driven, autonomous flow-switching schemes to facilitate parallel, long-term cellular studies of biorhythms [15] , [16] , [17] , [18] , [19] , [20] , emulating rhythmic stimulation such as those imposed by vascular flow and periodic hormone release. Similar to how low-voltage circuit design concepts were initially niche applications in the watch industry and later became indispensable in sophisticated electronics [21] , [22] , we believe that scalable low-pressure hydraulic circuit design concepts will have implications beyond our initial cell applications to become critical modules for a broad range of sophisticated microfluidic operations. As a model application that takes advantage of these capabilities, we systematically analyse endothelial cell elongation in response to different shear stresses and flow-switching periods. 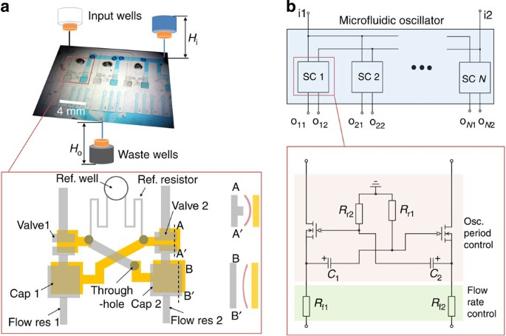Figure 2: Gravity-driven microfluidic oscillator. (a) An image of an oscillator array chip and schematic of one oscillator sub-circuit. Height difference between input wells and the oscillator chip applies a constant pressure on the oscillator sub-circuits. The inset shows the schematic of an oscillator sub-circuit, which consists of microfluidic component such as microfluidic resistors and capacitors. The microfluidic resistors are channels and the capacitors are chambers having elastomeric membranes. As shown in the cross-sections of the schematic, the valves and capacitors have a top layer (grey), a bottom chamber layer (dark yellow) and an elastomeric membrane (pink). The deflections of the membranes shown are what state the membranes would be in right after the opening of valve 2. Scale bar, 4 mm. (b) Circuit diagram of the oscillator. Each sub-circuit (SC) is connected in parallel. Sub-circuiti(i=1 toN) has two outlet ports (oi1and oi2). The inset presents the circuit diagram of the oscillator sub-circuit, which corresponds to the inset ofa.Cj(j=1, 2) is mechanical capacitance by an elastomeric membrane.RrjandRfjrepresent the fluidic resistances of reference resistors and flow resistors, respectively. Operation principles of oscillator sub-circuits Figure 2a shows an actual image of an oscillator array and a close-up schematic of one oscillator sub-circuit. As shown in the inset of Fig. 2a , the sub-circuit is composed of a three-layer structure including a thin-membrane middle layer, and top (grey colour) and bottom (dark-yellow colours) layers. These sub-circuits are comprised of microfluidic resistors (channels), capacitors, valves and a reference well. Microfluidic capacitors are chambers with elastomeric membranes that store pressure-related energy by membrane deformation. Valves are similar to the capacitors, except with much smaller membrane areas and a protrusion in the top chamber that leads to flow shut off. The reference well is a reservoir filled with liquid that is open to the atmosphere. The key design points are: to have the bottom chamber of the capacitor downstream of one valve connected to the bottom actuation chamber of the other valve, and to have reference resistors that connect the pair of interconnected capacitor–valve bottom chambers via a reference well (the insets of Fig. 2a,b ). Importantly, the fluid flowing through and out of the top chambers of the device remains separate from the bottom chamber fluid that connects the two valves to each other for actuation. In addition, owing to the reference well being open to atmosphere, the bottom actuation chamber pressures can increase and decrease somewhat independently from the upper flow-through chambers. Having an output pressure ( P o ) lower than the reference well pressure is also indispensable for being able to have valve closings [23] . Figure 2: Gravity-driven microfluidic oscillator. ( a ) An image of an oscillator array chip and schematic of one oscillator sub-circuit. Height difference between input wells and the oscillator chip applies a constant pressure on the oscillator sub-circuits. The inset shows the schematic of an oscillator sub-circuit, which consists of microfluidic component such as microfluidic resistors and capacitors. The microfluidic resistors are channels and the capacitors are chambers having elastomeric membranes. As shown in the cross-sections of the schematic, the valves and capacitors have a top layer (grey), a bottom chamber layer (dark yellow) and an elastomeric membrane (pink). The deflections of the membranes shown are what state the membranes would be in right after the opening of valve 2. Scale bar, 4 mm. ( b ) Circuit diagram of the oscillator. Each sub-circuit (SC) is connected in parallel. Sub-circuit i ( i =1 to N ) has two outlet ports (o i 1 and o i 2 ). The inset presents the circuit diagram of the oscillator sub-circuit, which corresponds to the inset of a . C j ( j =1, 2) is mechanical capacitance by an elastomeric membrane. R r j and R f j represent the fluidic resistances of reference resistors and flow resistors, respectively. Full size image How do the microhydraulic oscillator sub-circuits, described in this paper, trigger alternating valves to open and close with a constant input pressure ( P i )? Consider the top-side pressures of capacitors 1 and 2, P C1t and P C2t , respectively ( Fig. 3a ). When valve 1 opens, P C1t increases from ∼ P o to P i (−9 to 3 kPa, see Fig. 3b ), where for a given pressure head, the value of P C1t will depend on the relative values of capacitor 1’s upstream and downstream fluidic resistances ( Supplementary Fig. 1 ). Importantly, an increase in P C1t concomitantly increases the bottom pressure of capacitor 1 ( P C1b ), which is connected to valve 2, resulting in the closure of valve 2. While P C1b is high (9 kPa) immediately after valve 1 opens, the pressure gradually decreases over time as the pressurized fluid flows through the reference well and resistors towards capacitor 2 (inset ii of Fig. 3c ). As a result, while P C1b decreases P C2b increases. Once P C1b is low enough (1 kPa), valve 2 opens thereby abruptly raising P C2b and closing valve 1 (inset iii of Fig. 3c ). This process is repeated in an alternating manner resulting in oscillations. More detailed pressure relations, and valve-opening and -closing conditions are presented in Supplementary Fig. 2 . Note that unlike pneumatic valves, hydraulic valves require a relatively higher bottom pressure than top pressure of the valves to push the membrane into the closed position [7] , [23] . We achieve this condition by using a negative outlet pressure P o that reduces P C1t and P C2t and effectively helps valve closing by pulling the membrane into the closed position ( Supplementary Fig. 3 ). 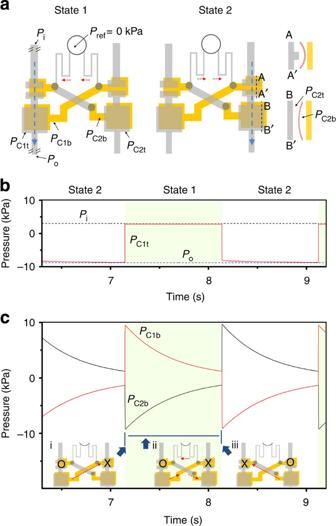Figure 3: Self-switching mechanism of the two valves of an oscillator sub-circuit. (a) Alternating opening and closing of the two valves. Valve 1 opens in state 1, and valve 2 opens in state 2. Note that when one valve opens, the other valve closes. Dotted blue arrows depict fluidic motion passing through the top side of the valves, and this motion becomes the output of the oscillator sub-circuit. Dotted red arrows illustrate the flows through reference channels, and this flow controls the switching period of the valves. Note that the two solution-flows represented by the blue and the red arrows do not mix owing to the membrane middle layer.PCitandPCib(i=1, 2) are the pressures of capacitori’s top and bottom, respectively. (b) Theoretical pressure profile ofPC1t.PiandPoare inlet and outlet pressures of the oscillator, respectively. (c) Theoretical pressure profiles ofPC1bandPC2b. Insets i, ii and iii illustrate the open (o) and close (x) states of the valves and fluid flows in the bottom layer (red arrows). Figure 3: Self-switching mechanism of the two valves of an oscillator sub-circuit. ( a ) Alternating opening and closing of the two valves. Valve 1 opens in state 1, and valve 2 opens in state 2. Note that when one valve opens, the other valve closes. Dotted blue arrows depict fluidic motion passing through the top side of the valves, and this motion becomes the output of the oscillator sub-circuit. Dotted red arrows illustrate the flows through reference channels, and this flow controls the switching period of the valves. Note that the two solution-flows represented by the blue and the red arrows do not mix owing to the membrane middle layer. P C i t and P C i b ( i =1, 2) are the pressures of capacitor i ’s top and bottom, respectively. ( b ) Theoretical pressure profile of P C1t . P i and P o are inlet and outlet pressures of the oscillator, respectively. ( c ) Theoretical pressure profiles of P C1b and P C2b . Insets i, ii and iii illustrate the open (o) and close (x) states of the valves and fluid flows in the bottom layer (red arrows). Full size image Independent control of oscillation periods and flow rates To control oscillation periods, we regulate the rate of change of P C1b and P C2b . As shown in Fig. 3c once valve 1 opens, the open state of valve 1 is maintained until P C1b decreases sufficiently. Thus, if P C1b drops slowly (or rapidly), valve 1 remains open longer (or shorter). Note that P ref is constant (0 kPa) and P C1t is also consistently at P i in the open state of valve 1. Between the two pressure points ( P ref and P C1t ), capacitor 1 and reference resistor 1 are serially connected. This makes the time constant for the open state of valve 1 to be R r1 C 1 ( Supplementary Fig. 4 ); similarly, the time constant for the open state of valve 2 is R r2 C 2 . Here, R r1 and R r2 are the fluidic resistances of reference resistors, and C 1 and C 2 are the mechanical capacitances of capacitor 1 and 2, respectively (see Fig. 2a,b ). We modify R r1 and R r2 across the sub-circuits to generate differential oscillation periods. On the other hand, output flow rate is determined by the fluidic resistance of flow resistors ( R f1 and R f2 , see Fig. 2b ). When valve 1 is open, P C1t is P i and outlet pressure is P o . Thus, the flow rate through flow resistor 1 is ( P i — P o )/ R f1 . Similarly, when valve 2 is open, the flow rate through flow resistor 2 is ( P i — P o )/ R f2 . Simply put, the micro-oscillator schematic can be broken into two functional compartments: one to determine the oscillation period and the other output flow rate, respectively, the light red-shaded and light green-shaded regions in Fig. 2b . Beyond being able to use a convenient gravity head as the pumping force, a fundamental utility of the oscillator array is that its sub-circuits can be connected in parallel, from the same gravity-driven pressure source, yet have completely independent oscillation frequencies without noise or crosstalk. To show the operational range and the parallel processing ability of our oscillator array, we constructed two distinct oscillator arrays: oscillator array A has fast oscillation periods and high flow rates, whereas oscillator array B has slow oscillation periods and low flow rates; see Supplementary Movies 1 and 2 . Detailed parameters of the two oscillator components are presented in Supplementary Fig. 5 . In sub-circuit A i ( i =1, 2, 3) of oscillator array A, flow resistor 1 ( Fig. 2a ) is connected to three downstream flow resistors (a i 1 , a i 2 , a i 3 ) that have three different fluidic resistances, respectively ( Fig. 4a ). As a result, sub-circuit A i generates three different fluidic pulse amplitudes through a i 1 , a i 2 and a i 3 ( Fig. 4b ). The flow rates of a i 1 , a i 2 and a i 3 are 5, 19 and 63 μl min −1 , respectively; sub-circuits A1 to A3 open their valves with periods of 0.4, 1.0 and 2.0 s, respectively. Sub-circuit A0 is simply a resistor, so it produces a constant output flow. 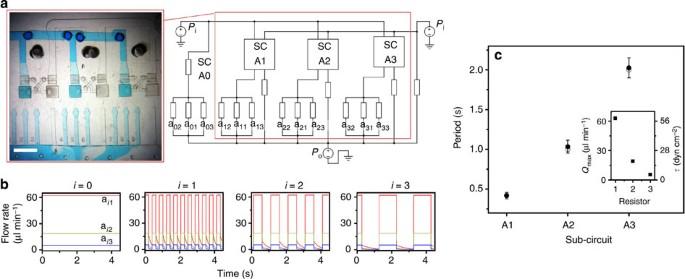Figure 4: Microfluidic oscillator array. (a) Photograph and circuit diagram of the multiple sub-circuits (SCs). Scale bar, 2 mm. (b) Theoretical flow profiles. Panels from left to right relate to flows in oscillator sub-circuit Ai(i=0–3). Flow profiles plotted in red (top), dark yellow (middle) and blue (bottom) are flows at resistors ai1, ai2and ai3, respectively, connected to oscillator sub-circuit Ai. (c) Performance of oscillators A. Filled and unfilled points are the experimental and theoretical results, respectively. The error bars are s.d. and were obtained from repeated measurements (n>20). The inset show the maximum flow rate (Qmax) and shear stress (τ) of resistors ai1, ai2and ai3ina. Figure 4c summarizes oscillation periods of the oscillators, and the inset of Fig. 4c presents the flow rates in a i 1 to a i 3 . Oscillator array B has four sub-circuits, which generate flow-oscillation periods of 10, 20, 66 and 119 min, respectively; two downstream flow resistors connected to each sub-circuit produces flow rates of 0.10 and 0.18 μl min −1 , respectively ( Supplementary Fig. 6 ). Figure 4: Microfluidic oscillator array. ( a ) Photograph and circuit diagram of the multiple sub-circuits (SCs). Scale bar, 2 mm. ( b ) Theoretical flow profiles. Panels from left to right relate to flows in oscillator sub-circuit A i ( i =0–3). Flow profiles plotted in red (top), dark yellow (middle) and blue (bottom) are flows at resistors a i 1 , a i 2 and a i 3 , respectively, connected to oscillator sub-circuit A i . ( c ) Performance of oscillators A. Filled and unfilled points are the experimental and theoretical results, respectively. The error bars are s.d. and were obtained from repeated measurements ( n >20). The inset show the maximum flow rate ( Q max ) and shear stress ( τ ) of resistors a i 1 , a i 2 and a i 3 in a . Full size image Cell morphology change under parallel shear stresses To demonstrate the utility of the oscillator arrays, we simultaneously evaluated the response of endothelial cells to multiple different levels of shear stress and periodic pulse in a single chip. The cells were seeded in resistors a i 1 to a i 3 of oscillator sub-circuits A i ( Fig. 4a ). The sub-circuits A1 to A3 generated periodic flow pulses of 0.5, 1 and 2.5 Hz, respectively, and sub-circuit A0 has a constant flow (0 Hz). The flows in resistors a i 1 , a i 2 and a i 3 applied shear stresses of 5, 18 and 58 dyn cm −2 , respectively, to the cells. 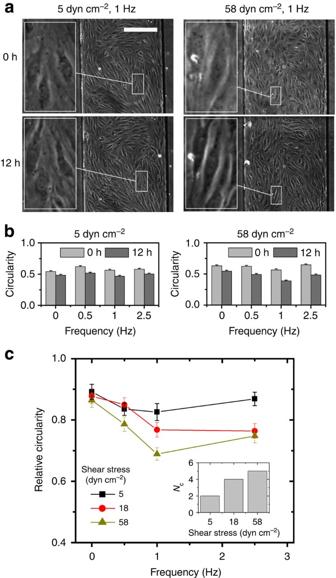Figure 5: Simultaneous on-chip testing of cell elongation response to shearing conditions. (a) Time-lapse micrographs showing endothelial cell elongation. Cells at 5 dyn cm−2show less elongation than those at 58 dyn cm−2. Pulse frequency is the same at 1 Hz. Scale bar, 200 μm. (b) Circularity of cells change significantly after a 12-h exposure to flows with shear stresses of 5 and 58 dyn cm−2at all pulse frequencies tested (P<0.001 by paired two-samplet-test at the 5% significance level). (c) Relative circularity at 12 h. The relative circularity is defined as the circularity at 12 h divided by the initial mean circularity at 0 h. The result is obtained from oscillator array A ofFig. 3a. Error bars ofbandcshow the s.e. (n=80). The inset shows the number (Nc) of frequency pairing combinations—out of the six possible combinations—with statistically significant differences (P<0.05) in relative circularity between them. Figure 5a compares time-lapse images of changes in the cell morphology at 5 versus 58 dyn cm −2 and 1 Hz pulsing for 12 h. The images show that the cells exposed to 58 dyn cm −2 are more elongated than those at 5 dyn cm −2 . To quantify the elongation, we use circularity that is defined as 4 πA/L p 2 . A is the area of the cell and L p is the perimeter of the cell. Shear stress has been demonstrated to elongate cells over time, consequently decreasing cell circularity, where circularity is 1 for a circle and 0 for a line. Figure 5b presents the change in cell elongation after 12 h at various levels of shear stress and pulsatile frequencies. The initial mean circularity of the cells in the channels varied from 0.57 to 0.63 (relative s.d.=6.4%). To systematically quantify the influence of various shear stress levels and pulse frequency on cell morphology, we use relative circularity, which is the circularity at 12 h divided by the initial mean circularity at 0 h. Lower relative circularity indicates cells are more elongated after 12 h. The results are summarized in Fig. 5c . Figure 5: Simultaneous on-chip testing of cell elongation response to shearing conditions. ( a ) Time-lapse micrographs showing endothelial cell elongation. Cells at 5 dyn cm −2 show less elongation than those at 58 dyn cm −2 . Pulse frequency is the same at 1 Hz. Scale bar, 200 μm. ( b ) Circularity of cells change significantly after a 12-h exposure to flows with shear stresses of 5 and 58 dyn cm −2 at all pulse frequencies tested ( P <0.001 by paired two-sample t -test at the 5% significance level). ( c ) Relative circularity at 12 h. The relative circularity is defined as the circularity at 12 h divided by the initial mean circularity at 0 h. The result is obtained from oscillator array A of Fig. 3a . Error bars of b and c show the s.e. ( n =80). The inset shows the number ( N c ) of frequency pairing combinations—out of the six possible combinations—with statistically significant differences ( P <0.05) in relative circularity between them. Full size image We found that as shear stress increased, frequency effects on circularity became more prominent. At each shear stress level, we used an independent two-sample t -test to compare two frequency conditions and identify statistically different cellular elongation. The four frequency conditions assessed produced six combinations of two frequency comparisons at each shear stress condition (the inset of Fig. 5c ). At 5 dyn cm −2 shearing, only two out of six combinations were significantly different. As the shear stress level increased from 18 to 58 dyn cm −2 , the combinations of significantly different pairs increased from 4 to 5 (see Supplementary Fig. 7 for more details). This result suggests that frequency effects on circularity increases with increasing shear rate. In addition, the trend at 18 dyn cm −2 is different from that at 5 and 58 dyn cm −2 . It is important to note that initial cell density varied by 23% in the flow resistors where cells were seeded: the highest and the lowest densities happened at the flow resistors where flow oscillation was 0.5 and 2.5 Hz of 18 dyn cm −2 , respectively. This density variation could also be of some influence on the observed relative circularity changes [24] . The angle of orientation, however, did not change significantly from 0 to 12 h ( Supplementary Fig. 8 ). This result agrees with previous studies [25] , [26] , in that cell alignment occurs more slowly than cell elongation. In addition, the cell density remained steady between 470 and 590 cells per mm 2 in all channels for the duration of the experiment, assuring that cell attachment was sufficient to resist the shear stress levels generated and that cell detachment was minimal. Analogy between electronic and hydraulic circuits provides a means to adapt the design of well-established electronic circuits to that of microfluidic circuits [1] , [2] . Interestingly, microhydraulic circuits that perform autonomous parallel operations driven by a constant water head alone, which also mimic parallel instruction-embedded electronic circuits, are conspicuously missing even when we also consider micropneumatic circuits in addition to microhydraulic circuits. This may in part be due to the prevalent use of macro-solenoid valves for time-varying pneumatic pressure inputs [4] , [5] , [13] . More fundamentally, gravity-driven, parallel switching operations cannot be accomplished in microhydraulic circuits simply by mimicking electronic circuit architectures, but must deal with and even take advantage of detailed features unique to hydraulic circuits and their components. Unlike electrical resistance that scales as radius ( r ) to the 1/ r 2 , fluidic resistance scales as 1/ r 4 . Consequently, fluidic resistance increases much more with decreasing device size when compared with electrical resistance. In addition, although electrical and fluidic resistances are linearly proportional to electrical resistivity ( ρ ) and fluidic viscosity ( μ ), respectively, ρ can be regulated in a wide range by selection of the electron-conducting material, whereas μ is fixed at a relatively high value for a given solution, regardless of what type of material is chosen for the channel. Specifically, ρ of copper and glass are 2 × 10 −8 and 1 × 10 9 Ohm m, respectively, but μ of water is 1 × 10 −3 Pa s. Thus, microfluidic circuits with digital circuit designs [3] , [4] , [5] , [6] , [7] , which inherently require massive serial integration of small components for logic operation, have issues with large pressure drops. Even with high-pressure actuation and pressure-gain methods [5] , such digital approaches can limit massively parallel flow control. The device described in this paper uses analogue circuit design concepts to minimize internal resistance for low-pressure operation: by reducing the number of components and lengths of resistive channels a fluid must flow through (blue arrow in Fig. 3a ); by separating the actuation fluid (red arrow in Fig. 3a ) from the flow-through fluid; and by parallel connection of the sub-circuits. Input pressures of microfluidic hydraulic digital circuits [5] , [13] are ∼ 100 kPa, which is equivalent to ∼ 10 m water head. In contrast, our device only needs a water head of 0.3–0.7 m (3–7 kPa). This low-pressure actuation by water head allows device actuation in a typical lab bench or incubator setting. The ability to use constant pressure inputs and convert them to parallel outputs is just as important as the ability to use low pressures. Unlike the constant-pressure oscillator described here, the input pressure of our previous constant-volumetric flow rate-driven oscillators fluctuates; see Fig. 2c of ref. 8 . Because the input pressures of the flow-driven oscillators connected in parallel fluctuates synchronously, parallel output flows with different flow-switching periods suffer severe crosstalk or are not possible. In contrast, the oscillator array in this report consists of parallel oscillator sub-circuits that switch with completely independent timing from each other. Theoretically, this enables unlimited number of the sub-circuits to work in parallel. The sub-circuits operate with a constant pressure that is provided through the height difference between the reservoirs and the devices. Importantly, we use a negative output pressure to satisfy the negative threshold pressure [23] required for our hydraulic valve closing. This is a feature of current hydraulic valves that differ from the switching-off characteristic of electronic transistors. One may wonder how these microhydraulic circuits compare with their pneumatic counterparts. Although a constant vacuum-driven ring oscillator can generate clock signals for microfluidic pneumatic digital logic circuits [27] , the pneumatic approaches still require other temporally programmed pressure-input pulses to control parallel outputs [4] , thereby the use of constant pressure input alone for such circuits has not been demonstrated. Digital circuit design concepts also require significantly larger number of components compared with analogue circuit designs of similar functions (see Supplementary Fig. 9 ), leading to practical fabrication challenges as well as pressure drop challenges. Finally, unlike microhydraulic circuits where the assay solutions are directly manipulated within the circuit, pneumatic logic circuits require that liquid solutions be manipulated indirectly through a completely separate network of channels. As an application, we studied cell morphology change within hydraulic oscillator arrays that generate various flow rates and oscillation periods in parallel channels. These devices facilitated a systematic study of the combinatorial effects of shear stress levels and flow-oscillation frequencies on endothelial cell elongation. Previously, a microfluidic approach using Braille pins [26] was applied to endothelial shearing; however, this work did not independently control flow rate and pulse frequency, because the pin actuation frequency simultaneously affect both parameters, thereby limiting the systematic study of flow rate and pulse frequency on cell morphology. Other devices [28] , [29] , [30] , [31] also have not tested different flow rates and pulse frequencies in parallel channels, at least partially because of the substantial automation required for parallel pulsed shear experiments. Thus, previous devices have been limited in simultaneous screening across a broad range of shear stresses [26] , [28] and pulse frequencies [29] , [30] , [31] . While the achieved gravity-driven flow rates of 0.1–63 μl min −1 are somewhat limited, it is important to note that this range covers most of the range of flows important for biomedical microfluidics. At the lower end, 0.02 dyn cm −2 is ideal for culture of delicate cells such as neurons or assays that require gentle flow. The higher flow rates provide shear stresses estimated to be up to 58 dyn cm −2 in our channels enabling exposure of endothelial cells to the higher range of shear stress experienced by cells physiologically. Also, wide oscillation periods (0.4 s–2 h) implemented in our oscillator could be used to study various biological rhythms such as periodic shearing by heart beating, periodic hormone secretion and calcium oscillation [15] , [20] . Importantly, such applications would be available in an incubator setting owing to the constant low-pressure actuation by a water head. While our work focused on cellular applications, the design principles for constant-pressure-driven, parallel instruction-embedded devices should be applicable for a broad range of applications where microhydraulic devices with multiple independent and autonomous sub-circuits are required. Device fabrication We fabricated the oscillators using soft lithography [32] . In master molds, the features of reference resistors were fabricated first by a deep reactive ion etching of a Si wafer and then the other features by SU-8 photolithography. We silanized the master mold with tridecafluoro-1,1,2,2-tetrahydrooctyl-1-trichlorosilane (United Chemical Technologies) in a desiccator, and continued it for 4 h to promote facile demolding of casting material. The casting material was made from poly(dimethylsiloxane) prepolymer and curing agent (Sylgard 184, Dow Corning) at a 10:1 ratio. The oscillators for device operation consisted of three layers: the top and the bottom layers having the features of microfluidic components were cast against the master molds with a curing temperature of 60 °C overnight. The middle layer is a membrane layer (40 and 30 μm-thicknesses for oscillators A and B, respectively), and was spin-coated on a silanized glass slide, and then cured at 120 °C for 20 min. Detailed bonding process is shown in supporting information of ref. 10 . Computational simulation and flow-oscillation experiment For developing the theoretical model of the oscillator, we used a commercial software (PLECS, Plexim GmbH). Detailed circuit diagram of the model and parameters of each microfluidic component are presented in Supplementary Fig. 5 . For the flow visualization, we mixed a blue food dye. To facilitate the introduction of working solutions, the device was put in a vacuum for 5 min and then in ambient pressure for 40 min. We measured the pressures of device inlet and connection tube outlet from height difference between the reservoirs and the oscillator, and the connection tube outlet and the oscillator, respectively. Working solutions were deionized water. Maximum flow rate ( Q max ) was calculated by Poiseuille’s law, Q max =Δ p / R . Here, Δ p is the pressure difference between device inlet and connection tube outlet, and R is a fluidic resistance between the inlet and outlet pressures. Shear stress ( τ ) was calculated by τ =6μ Q max /( wh 2 ), where μ is the dynamic viscosity and w and h are the width and height of a flow resistor, respectively. Cell culture and imaging For the shear flow experiment, we used human umbilical vein endothelial cell (HUVECs). HUVECs were cultured in endothelial cell growth media (CC-3162, Lonza) under 37 °C, 5% CO 2 on T-25 flasks. Then, 0.25% Trypsin/EDTA (Gibco) was used to detach cells from the flasks. For the cell seeding in the flow resistors, laminin (10 μg ml −1 in PBS) was injected along the flow resistors and incubated in a CO 2 incubator for 1 h to coat the resistor surface. Then, the laminin solution was carefully washed with PBS, and cells were injected into the resistors and maintained with DMEM under 37 °C, 5% CO 2 for a day. For the cell shearing, we used CO 2 -independent media (Invitrogen) with growth factors (CC-4176, Lonza), and the oscillator temperature was maintained at 36±1 °C. Cell images were acquired every 2 h. The program MetaMorph (Molecular Devices) was used for image acquisition, and the program ImageJ (NIH) was used to measure circularity and angle of orientation. How to cite this article: Kim, S.-J. et al. Multiple independent autonomous hydraulic oscillators driven by a common gravity head. Nat. Commun. 6:7301 doi: 10.1038/ncomms8301 (2015).